Valley-selective circular dichroism of monolayer molybdenum disulphide A two-dimensional honeycomb lattice harbours a pair of inequivalent valleys in the k -space electronic structure, in the vicinities of the vertices of a hexagonal Brillouin zone, K ± . It is particularly appealing to exploit this emergent degree of freedom of charge carriers, in what is termed 'valleytronics'. The physics of valleys mimics that of spin, and will make possible devices, analogous to spintronics, such as valley filter and valve, and optoelectronic Hall devices, all very promising for next-generation electronics. The key challenge lies with achieving valley polarization, of which a convincing demonstration in a two-dimensional honeycomb structure remains evasive. Here we show, using first principles calculations, that monolayer molybdenum disulphide is an ideal material for valleytronics, for which valley polarization is achievable via valley-selective circular dichroism arising from its unique symmetry. We also provide experimental evidence by measuring the circularly polarized photoluminescence on monolayer molybdenum disulphide, which shows up to 50% polarization. A non-equilibrium charge carrier imbalance between valleys is the key to creating valleytronic devices [1] , [2] , [3] , [4] , [5] , [6] , [7] , [8] , [9] . The principal mechanism invoked in this context is circularly polarized optical excitation [3] , [4] . In this approach, the two valleys absorb left- and right-handed photons differently, a phenomenon referred to as circular dichroism (CD). An essential condition for valley-selective CD in a honeycomb lattice is the absence of a centre of inversion. In the case of graphene, it was suggested that by interacting graphene with a substrate such that the centre of inversion can be obliterated, whereupon a gap opens up in each valley [10] , [11] . This strategy, however, is quite challenging experimentally. And even in its eventual realization, there can only be a gentle perturbation to graphene via the weak covalent coupling at large van der Waals separations from the substrate [11] . Since its first isolation [12] , [13] , monolayer molybdenum disulphide (MoS 2 ) has attracted immense attention. Many measurements have been performed to characterize the optical and transport properties of this material [12] , [13] , [14] , [15] , [16] . In monolayer MoS 2 , two layers of sulphur atoms in a two-dimensional hexagonal lattice are stacked over each other in an eclipsed fashion. Each Mo sits in the centre of a trigonal prismatic cage formed by six sulphur atoms ( Fig. 1a ). Quite remarkably in the context of current discussion, the natural stable structure of free-standing monolayer MoS 2 is a honeycomb lattice with inequivalent bipartite colouring, breaking the inversion symmetry ( Fig. 1b ). 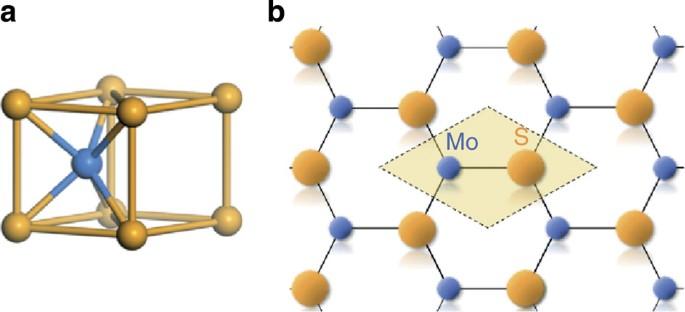Figure 1: The crystal structure of monolayer MoS2. (a) Coordination environment of Mo (blue sphere) in the structure. Sulphur is shown as golden spheres. (b) A top view of the monolayer MoS2lattice, emphasizing the connection to a honeycomb lattice. In our calculations, we used an optimized structure at the level of local density approximation in density functional theory. The shaded region bounded by dashed lines corresponds to one primitive cell. The unit cell parameter isa=3.12 Å, and the vertical separation between sulphur layers is 3.11 Å. Figure 1: The crystal structure of monolayer MoS 2 . ( a ) Coordination environment of Mo (blue sphere) in the structure. Sulphur is shown as golden spheres. ( b ) A top view of the monolayer MoS 2 lattice, emphasizing the connection to a honeycomb lattice. In our calculations, we used an optimized structure at the level of local density approximation in density functional theory. The shaded region bounded by dashed lines corresponds to one primitive cell. The unit cell parameter is a =3.12 Å, and the vertical separation between sulphur layers is 3.11 Å. Full size image While bulk MoS 2 has an indirect bandgap, interestingly, when thinned to the monolayer limit, the material acquires direct bandgaps located exactly at the corners of the Brillouin zone. Indeed, with its 1.8 eV direct bandgap and unique two-dimensional structure embracing the high-symmetry valleys, monolayer MoS 2 has much to offer in the exploration of novel electronic and optoelectronic devices and the associated physics (as compared with boron nitride, which has a bandgap of about 6.0 eV in the ultraviolet regime). It is quite natural to question whether it is possible to achieve valley-selective CD in this semiconducting atomic membrane, which will endow electrons in this material the valley degree of freedom, in addition to charge and spin that have been routinely explored in conventional device physics. We show here using ab initio numerical simulation and experimental micro-photoluminescence that monolayer MoS 2 possesses near-perfect valley-selective CD, a property rooted in its bulk symmetry and very much conducive to optoelectronic valley polarization needed for valleytronics. Degree of circular polarization The key quantity to assess is, therefore, the k -resolved degree of optical polarization, η ( k ), between the top of the valence bands and the bottom of the conduction bands [4] This quantity is the difference between the absorption of left- and right-handed lights (±), normalized by total absorption, at each k -point and evaluated between the top of the valence bands ( v ) and the bottom of conduction bands ( c ). The band structure of monolayer MoS 2 is shown in Fig. 2a . The dependence on the transition energy, , is implicit through k . Here, the transition matrix element of circular polarization is . The interband matrix elements, , are evaluated using the density functional perturbation theory, within the local-density approximation [17] , as implemented in VASP [18] . Spin-orbit coupling is not included in our calculations [19] , [20] . Briefly, a planewave basis set is employed at a cutoff energy 600 eV, and a total of 80 bands are included to ensure convergence of all computed quantities. A very dense k -point mesh (15129 grid points) over the reducible hexagonal Brillouin zone is sampled in our calculations. 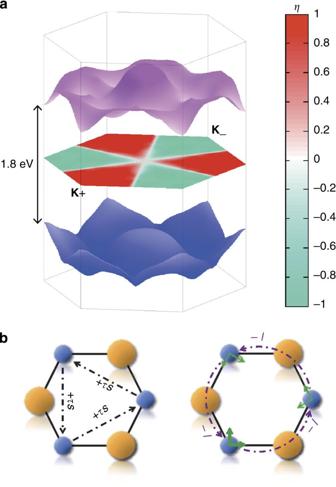Figure 2: Valley-selective CD of monolayer MoS2. (a) Top valence band (blue) and bottom conduction band (pink). The centre hexagon is the Brillouin zone colour-coded by the degree of circular polarization,η(k), as defined in the text. The vector connectingK+andK−is perpendicular to Mo-S bond in the crystal structure inFig. 1b. (b) Schematic of phase winding on the MoS2lattice that gives rise to the chiral optical selectivity. Left panel: the contribution to phase winding from the Bloch lattice phase, whereτ=±1 is the valley index, ands=1,2 corresponding to the S and Mo sites (isospin index). Right panel: the phase winding under a threefold rotation. The green axes indicate the rotation of local atomic coordinates that leads to the azimuth dissynchronization. Figure 2: Valley-selective CD of monolayer MoS 2 . ( a ) Top valence band (blue) and bottom conduction band (pink). The centre hexagon is the Brillouin zone colour-coded by the degree of circular polarization, η ( k ), as defined in the text. The vector connecting K + and K − is perpendicular to Mo-S bond in the crystal structure in Fig. 1b . ( b ) Schematic of phase winding on the MoS 2 lattice that gives rise to the chiral optical selectivity. Left panel: the contribution to phase winding from the Bloch lattice phase, where τ =±1 is the valley index, and s =1,2 corresponding to the S and Mo sites (isospin index). Right panel: the phase winding under a threefold rotation. The green axes indicate the rotation of local atomic coordinates that leads to the azimuth dissynchronization. Full size image As shown in Fig. 2a , chiral absorption selectivity is indeed exact at K ± with η =±1. The contrast in the chiral absorptivities between the valleys owes its origin to the symmetry of both lattice and local atomic orbitals, which is quite different from the gapped graphene case [4] . A band state relevant to the optical excitation originates from local atomic states, bearing different orbital magnetic quantum numbers, l , or more generally as Wannier function, where ( r , θ , ) are the standard spherical coordinates taking the z -direction perpendicular to the plane of MoS 2 . In the case of monolayer MoS 2 , the states at the top of the valence bands involve only and d xy on Mo, and p x and p y states on S. At K + , the d -states on Mo hybridize as (l=+2) to interact with ( l =+1). At K − , the d -states on Mo hybridize as ( l =−2) to interact with ( l =−1). At the bottom of the conduction band, mainly state on Mo ( l =0) is involved with a minor contribution from the p -orbitals of S. These atomic orbitals form such linear combinations in accordance with the D 3 h point group symmetry and the lattice translational symmetry. Microscopic chiral selection rule The optical selection rule is rooted in the phase winding of the Bloch states under rotational symmetry, threefold rotation ( ) in this case. Given the symmetry-adapted linear combinations of the atomic orbitals, the azimuthal phase associated with the threefold rotation at K ± is readily calculable, and where v and c correspond to the valence and conduction band extrema, respectively. Notice, however, the phase winding associated with the rotation has two distinct contributions, as schematically illustrated in Fig. 2b . The first comes from the Bloch phase shift in stepping from one lattice site to a next, as in the case of gapped graphene [3] . The second phase factor arises as a consequence of dissynchronization of the azimuthal phase (associated with the magnetic quantum number, l ) concomitant with rotation of local atomic coordinates (green axes in Fig. 2b ). Now the chiral optical selectivity of the valleys can be deduced. The bottom of the conduction bands at the valleys, dominated by the l =0 d -states on Mo, bears an overall azimuthal quantum number m ± =±1, at K ± . At the top of the valence bands, m ± =0. Then for an optical transition at K ± , the angular momentum selection rule indicates that Δ m ± =±1, corresponding to the absorption of left- and right-handed photons. Therefore, our density functional perturbation theory results concerning the close neighbourhood of the valleys, which is most important to the proposed optical valley polarization, are in fact ensured by the symmetry of the material. There is an important distinction, compared with gapped graphene, in the microscopic origin of chiral optical selection rule; that is, the selectivity arises directly from the local relative azimuthal phase of the atomic orbitals, in contrast to the sublattice-dependent Bloch phase winding in the case of gapped graphene [3] . The bonding of the electronic states in MoS 2 across the gap is also considerably more complex, exhibiting richer possibilities of variation owing to the symmetry of local atomic states. Remarkably, the selectivity is nearly perfect over the entire valleys, and only changes sign rapidly across valley boundaries ( Fig. 2a ). This is to say, the entire valley K + absorbs almost purely left-handed photons, whereas the entire valley K − purely right-handed. The perfect intrinsic valley-constrasting CD is very much conducive to optical polarization of the valleys. When a left (right)-handed light is shone over the sample, a non-equilibrium state will be created where the charge carrier population resides mostly in K + ( K − ) valley (valley polarization). Circularly polarized photoluminescence To further confirm our theoretical and numerical results, we have also performed experimental circularly polarized photoluminescence (PL) measurements on monolayer MoS 2 . The polarization of PL is an indication of how good the chiral optical selectivity is, and of how well the valley identity of charge carriers is preserved before recombination. Fig. 3a,b show the samples on which our experiments are performed. The monolayer region is identified by micro-PL at 300 K ( Fig. 3c ), as in a monolayer sample displays a single PL peak at 1.82 eV, while multi-layer samples show an additional peak at lower energies [12] . In Fig. 3d , we show the intensities of the luminescence with σ + (left-handed) and σ − (right-handed) polarizations at low temperature (83 K), under a σ + irradiation at wavelength 633 nm (see Methods). In agreement with our prediction, the luminescence indeed exhibits a substantial circular polarization ( η ~50%) at the PL peak. 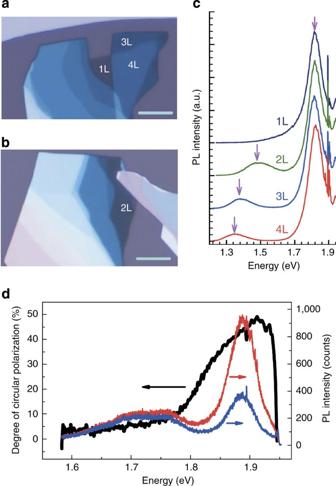Figure 3: Experimental measurements of circularly polarized PL of monolayer MoS2. (a) and (b) Optical images of one-to-four-layer samples (1L to 4L) on which micro-PL is performed, where 1L, 2L, 3L and 4L regions are labelled. The scale bars correspond to 5 microns. (c) Micro-PL of monolayer and few-layer MoS2at 300 K. Each spectrum is normalized by its maximum intensity. Arrows indicate the lowest-energy peak of each spectrum. (d) Circularly polarized micro-PL of monolayer MoS2at 83 K, along with the degree of circular polarization of the PL spectra. The red and blue curves correspond to the intensities ofσ+andσ−polarizations, respectively, in the luminescence spectrum. The black curve is the net degree of polarization. Figure 3: Experimental measurements of circularly polarized PL of monolayer MoS 2 . ( a ) and ( b ) Optical images of one-to-four-layer samples (1L to 4L) on which micro-PL is performed, where 1L, 2L, 3L and 4L regions are labelled. The scale bars correspond to 5 microns. ( c ) Micro-PL of monolayer and few-layer MoS 2 at 300 K. Each spectrum is normalized by its maximum intensity. Arrows indicate the lowest-energy peak of each spectrum. ( d ) Circularly polarized micro-PL of monolayer MoS 2 at 83 K, along with the degree of circular polarization of the PL spectra. The red and blue curves correspond to the intensities of σ + and σ − polarizations, respectively, in the luminescence spectrum. The black curve is the net degree of polarization. Full size image The experimentally measured polarization of the PL is considerably larger than spin-related polarization in other widely studied materials such as GaAs, but smaller than the expected value from ab initio simulation ( η≥ 0.98 for the energy of the incident light). There are two important timescales in the valley-optical processes: valley lifetime, τ v , and recombination time, , in which subscripts r and nr refer to radiative and non-radiative recombinations (via, for example, the substrate), respectively. The value of polarization of the experimental PL, η PL , can be deduced from standard rate equations for the steady-state process, where 1− δ is selectivity in the initial excitation (including possible intervalley generation), and η the theoretical degree of circular polarization. In the lowest order description of the kinetic processes, we have δ = δ imp + δ ph to account for impurity/defects/substrate- and phonon-assisted excitation and recombination in which the valleys are coupled by the momentum components of the scatterers. Consequently, the less-than-perfect circular polarization observed in the experimental PL is ascribable to inevitable intervalley processes, or relatively large ratio between valley lifetime and recombination time, τ / τ v . Measurements of PL circular polarization on high-quality, clean samples at very low temperatures (minimizing δ ) will allow the extraction of τ / τ v . Moreover, it is interesting to assess the role of non-radiative relaxation of carriers, which can be induced by substrate [12] and defects. Now that we have established the valley-selective CD in monolayer MoS 2 with ensuing non-equilibrium valley polarization, it is also interesting to inspect the Berry curvature, , which, if present, has crucial influence on the electronic transport properties. Berry curvature enters into the semiclassical wavepacket dynamics via an anomalous velocity perpendicular to the applied electric field (~ E × Ω n ( k )), in addition to the usual group velocity of a Bloch band state [21] , [22] . Although Berry curvature is not exactly a ground-state property, it can be evaluated quite accurately for the Kohn-Sham one-particle states [23] , [24] . The presence of non-vanishing Berry curvature is possible in the non-centrosymmetric honeycomb lattice [3] . In Fig. 4 , we plot the Berry curvature, along the K − −Γ− K + path. Because the system has time-reversal symmetry and not inversion symmetry, Ω n,z ( k ) is an odd function in k with generally non-zero values, as expected. The charge carriers' anomalous velocities acquire opposite signs in the two valleys, exactly cancelling each other's contribution to the transverse current. At equilibrium, freestanding monolayer MoS 2 will not exhibit valley Hall effect, as expected. At K ± , the Berry curvatures do not have the particle-hole symmetry. This is a clear indication that the physics of MoS 2 cannot be fully captured by a minimalistic two-band model, as is distinct from the case of gapped graphene. 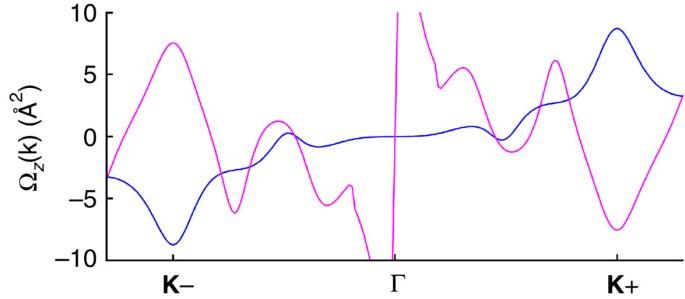Figure 4: Berry curvature, Ωn,z(k), of bands across the bandgap. The blue curve corresponds to the top of valence bands. The red curve corresponds to the bottom of conduction bands. The Berry curvatures of the states along theK−−Γ−K+path of the Brillouin zone are plotted. The value of Berry curvature is large for the conduction band at the zone centre, where bands are degenerate. Figure 4: Berry curvature, Ω n,z ( k ), of bands across the bandgap. The blue curve corresponds to the top of valence bands. The red curve corresponds to the bottom of conduction bands. The Berry curvatures of the states along the K − −Γ− K + path of the Brillouin zone are plotted. The value of Berry curvature is large for the conduction band at the zone centre, where bands are degenerate. Full size image On the bais of our theoretical and experimental results, a few further experiments are quite compelling. When valley polarization is induced by, say, valley-selective CD, only one valley has non-vanishing charge carrier population (ideally, assuming the absence of intervalley scattering). This can then lead to the Hall effect and magnetization without an applied magnetic field [4] . The Berry curvature across the band edges near K ± is most relevant to photo-excited charge carriers. We see that, at the band edges, both conduction and valence bands display significant Berry curvature with opposite signs. Consequently, when electrons and holes are generated by a circularly polarized irradiation, both types of charge carriers have an intrinsic concurrent contribution to the Hall conductivity or magnetization. Moreover, a time-resolved PL measurement will also be an interesting experiment for revealing the valley lifetime, analogous to the spin lifetime in spintronics. In closing, we also would like to point out that MoS 2 is but one of the many transition metal dichalcogenides, MX 2 , where M=Mo, W, and X=S, Se. They all have identical crystal structure and are similar electronically. These compounds, once available in monolayer form, will provide a chemically rich family of semiconducting atomic membranes for exploring the valley physics, as we have demonstrated here for MoS 2 . In addition, there is considerable spin-orbit coupling in these systems [19] , and the valley and spin dependent physics in the neighbourhood of K points in MoX 2 monolayers is discussed in a recent theoretical work [20] . The evaluation of optical selecivity and Berry curvature at higher level theories to address the many-body nature of the excited states is also an important future direction. Sample preparation MoS 2 flakes consisting of 1–4 layers (L) are obtained by micro-mechanical cleavage of a natural bulk MoS 2 crystal (SPI Supplies, USA) on a Si/90 nm SiO 2 substrate. The number of layers is identified by optical contrast and PL spectroscopy. Circularly polarized micro-PL Optical contrast and micro-PL are performed in a backscattering geometry using a Jobin-Yvon HR800 Raman system equipped with a liquid-nitrogen-cooled charge-coupled detector. The optical excitation wavelength is 633 nm from a HeNe laser. The laser beam passes through a Soleil Babinet Compensator to generate a circularly polarized light. The polarization is set to σ + , and the PL polarization σ + or σ − is analysed by a quarter-wave plate placed in front of a fixed Glan–Thomson linear polarizer. The whole set-up provides a rejection ratio better than 5% in σ + and σ − configuration over the spectral range of interest. The excitation power of 50 μW is used to avoid sample heating. We use a normal ×100 objective with numerical aperture =0.90 for optical contrast and PL measurement at room temperature ( Fig. 3c ). A long-working-distance ×50 objective is used for PL measurement at low temperature ( Fig. 3d ). The sample temperature was controlled by a programmable hot stage THMS600 from Linkam Scientific Instruments. How to cite this article: Cao, T. et al . Valley-selective circular dichroism of monolayer molybdenum disulphide. Nat. Commun. 3:887 doi: 10.1038/ncomms1882 (2012).